Switching action modes of miR408-5p mediates auxin signaling in rice 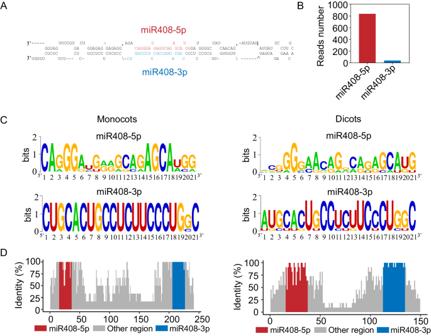Fig. 1: Identification and conservation analysis of miR408-5p and miR408-3p in plants. ASecondary structure ofMIR408precursor in rice. Red sequences indicate mature miR408-5p while blue sequences indicate mature miR408-3p.BReads number of rice miR408-5p and miR408-3p in miRbase.CSequences of miR408-5p and miR408-3p in monocots and dicots shown by seqlogo.DThe evolutionary analysis ofMIR408precursor in monocots and dicots. The precursor sequence data are collected from miRbase website. Red and blue bars denote miR408-5p and miR408-3p regions, respectively.X-axis means the length ofMIR408precursor andy-axis indicates the value of identical sequences. Source data underlying (B) are provided as a Source Data file. MicroRNAs (miRNAs) play fundamental roles in many developmental and physiological processes in eukaryotes. MiRNAs in plants generally regulate their targets via either mRNA cleavage or translation repression; however, which approach plays a major role and whether these two function modes can shift remains elusive. Here, we identify a miRNA, miR408-5p that regulates AUXIN/INDOLE ACETIC ACID 30 ( IAA30 ), a critical repressor in the auxin pathway via switching action modes in rice. We find that miR408-5p usually inhibits IAA30 protein translation, but in a high auxin environment, it promotes the decay of IAA30 mRNA when it is overproduced. We further demonstrate that IDEAL PLANT ARCHITECTURE1 (IPA1), an SPL transcription factor regulated by miR156, mediates leaf inclination through association with miR408-5p precursor promoter. We finally show that the miR156-IPA1-miR408-5p-IAA30 module could be controlled by miR393, which silences auxin receptors. Together, our results define an alternative auxin transduction signaling pathway in rice that involves the switching of function modes by miR408-5p, which contributes to a better understanding of the action machinery as well as the cooperative network of miRNAs in plants. MicroRNAs (miRNAs) are 20–24 nucleotide (nt) small RNAs that play fundamental roles in the regulation of gene expressions in eukaryotes. The primary miRNA unit in both animal and plants is typically transcribed by RNA polymerase II and forms a stem-loop transcript [1] . This hairpin precursor (pre-miRNA) is subsequently excised as an RNA duplex by an RNase III enzyme, Dicer or Dicer-like (DCL) protein, and generates two strands, one strand designated as miRNA*, which is degraded, while the other strand is called miRNA that enters ARGONAUTE (AGO)-mediated RNA-induced silencing complexes, where it scans complementary sequences and execute its functions [2] . Plant miRNAs have been thought to predominantly slice transcripts due to their strict base-pairing with targets in contrast to animal miRNAs, which appear to be imperfectly matched with and mediate targets through translation inhibition. A couple of studies have shown that certain targets of miRNAs exhibit discrepancies between their transcripts and protein products, indicating that plant miRNAs have the capability to suppress target translation in addition to transcript degradation [3] , [4] , [5] , [6] , [7] . Furthermore, several factors that are specific to miRNA-entailed translational repression have been genetically characterized [3] , [8] , [9] , [10] , [11] , [12] , supporting the notion that two action modes of miRNAs can be separated in plants. Nevertheless, because mRNA cleavage and protein translation inhibition seem to have similar sequence matching requirements between miRNA and targets in plants, and the decrease of mRNA gives rise to a reduction of protein, it is difficult to determine which regulatory mode of miRNA is more important, and whether miRNA can swap the two modes of target regulation is largely elusive [13] , [14] . Phytohormones play pivotal roles in almost all aspects of plant growth. As a key mediator of plant development, auxin is perceived by the receptors TRANSPORT INHIBITOR RESPONSE1 (TIR1)/AUXIN SIGNALING F BOX PROTEINS (AFBs), which leads to the activation of AUXIN RESPONSE FACTORS (ARFs) transcriptional factors through proteasomal degradation of a set of AUX/ INDOLE ACETIC ACID (IAA) family proteins [15] . Several miRNAs have been revealed to play roles in regulation of major steps in auxin signaling. For example, miR393, a conserved miRNA in diverse plants, cleaves TIR1/AFB transcripts and triggers the biogenesis of phased secondary siRNAs (phasiRNAs) to keep the homeostasis of Auxin cascade [16] , [17] , [18] . Thus, the networks involving miRNAs, phasiRNAs, mRNAs and proteins contribute to the robustness and flexibility to growth and development influenced by plant hormones. One of the greatest challenges in crop improvement is that the trade-off between introducing a desirable trait in a new variety and potentially missing other beneficial characteristics [19] . However, miR156, a conserved small RNA molecule found in multiple plants, has emerged as an ideal for manipulating various important agronomic features through regulating a class of SQUAMOSA PROMOTER BINDING PROTEIN-LIKE (SPL) transcription factors [20] , [21] , [22] , [23] , [24] . Similarly, miR408 is also recently implicated as a promising candidate for crop improvement, since overexpression of miRNA408 has been shown to increase growth, photosynthesis and grain yield by down-regulating UCLACYANIN 8 ( UCL8 ), a phytocyanin family gene, thereby impairing copper homeostasis in rice [25] , [26] , [27] . In previous study, we demonstrated that miRNA precursors in rice have the ability to generate multiple mature miRNAs simultaneously through the cooperative actions of different DCLs [28] . Similarly, MIR408 , which is annotated in miRbase, is capable to produce two mature miRNAs, namely miR408-5p and miR408-3p (previously designated as miR408) in rice. Although the role of miR408-3p in growth and tolerance to stresses is clear, the targets and effects of miR408-5p on rice performance remain unknown. Here, we illustrated that miR408-5p is involved in auxin signaling in rice. Most strikingly, our finding reveals that miR408-5p usually inhibits target protein translation, but switches to mediate target mRNA cleavage when it is over-accumulated. Furthermore, we found that miR393 and miR156, two conserved miRNAs in plants, could hierarchically act with miR408-5p in the rice auxin pathway to control leaf inclination. Together, our results define a novel auxin transduction signaling pathway that is mediated by switching of function modes of miR408-5p. miR408-5p is abundant in rice The rice genome contains a single MIR408 locus, and the pre-miR408 has been annotated to generate two mature miRNAs, miR408-5p and miR408-3p, from each arm of the precursor (Fig. 1A ). It is clear that miR408-3p is a conserved miRNA among different plant species and is therefore considered to be more abundant than miR408-5p; however, when we checked their abundance in miRbase [29] , we unexpectedly found that the copy reads of miR408-5p were higher than those of miR408-3p in rice (Fig. 1B ). We further calculated the normalized expression levels of miR408-5p and miR408-3p using PmiRExAt, a plant miRNA expression atlas database [30] , and found a comparable quantity of miR408-5p to that of miR408-3p in specific tissues, such as leaf and callus, despite the overall lower accumulations of miR408-5p compared to miR408-3p in rice (Fig. S1A, B ). Nevertheless, when we examined other rice miRNA precursors that can generate two mature miRNAs, we consistently observed significantly lower expression levels of non-conserved miRNAs than the conserved ones in all cases (Fig. S1A, B ). These results suggest that miR408-5p is an abundant miRNA in rice and may therefore possess biological importance. Fig. 1: Identification and conservation analysis of miR408-5p and miR408-3p in plants. A Secondary structure of MIR408 precursor in rice. Red sequences indicate mature miR408-5p while blue sequences indicate mature miR408-3p. B Reads number of rice miR408-5p and miR408-3p in miRbase. C Sequences of miR408-5p and miR408-3p in monocots and dicots shown by seqlogo. D The evolutionary analysis of MIR408 precursor in monocots and dicots. The precursor sequence data are collected from miRbase website. Red and blue bars denote miR408-5p and miR408-3p regions, respectively. X -axis means the length of MIR408 precursor and y -axis indicates the value of identical sequences. Source data underlying ( B ) are provided as a Source Data file. Full size image The presence of overlapping sequences between rice miR408-5p with miR408-3p* promoted us to explore the evolutionary history of these two miRNAs generated from miR408 precursor. The higher number of identical sequences in miR408-3p compared to miR408-5p suggested that miR408-3p is more conserved than miR408-5p (Fig. 1C, D ). Interestingly, we found that both variations of miR408-5p and miR408-3p were a slightly higher in dicotyledons than in monocotyledons (Fig. 1C, D ), implicating a potentially faster evolution of MIR408 genes in dicots than in monocots. Moreover, we observed that the middle region of the MIR408 stem-loop structure was significantly longer in monocots compared to dicots (Fig. 1D ), and whether this difference contribute to the higher conversation of the mature miRNAs in monocots than that in dicots remains to be further determined. IAA30 is targeted by miR408-5p in rice To investigate the potential function of miR408-5p in rice, we predicted its target genes by PsRobot, a widely used small RNA analysis toolbox [31] . Interestingly, among the predicted targets using strict parameters, we identified an Auxin-responsive Aux/IAA gene family member, IAA30 , with a potential target site located at the 3′Untranslated Region (UTR) (Fig. 2A ). However, when we relaxed the computational prediction criteria, three Aux/IAA members, IAA11 , IAA19 and IAA30 , were estimated as miR408-5p targets (Fig. S2A ). Among them, IAA30 had the highest complementarity to miR408-5p, while IAA19 and IAA11 harbored more bulges and mispairings with miR408-5p (Fig. S2A ), implying that IAA30 is more likely to be the genuine target of miR408-5p. Fig. 2: miR408-5p targets IAA30 and is induced by auxin in rice. A Gene structure of IAA30 and alignments of miR408-5p with target sites in IAA30 3′UTR and mutant 3′UTR (m3′UTR). B Validation of IAA30 as miR408-5p target through transient expression analysis in N. benthamiana leaves. Left: The constructs in A. tumefaciens transiently introduced in N. benthamiana leaves. Middle: Representative photograph of firefly luciferase fluorescence signals when the indicated construct combinations were introduced in N. benthamiana leaves. Right: Relative reporter activity in N. benthamiana leaves expressing the indicated construct combinations. Error bars indicate SD (Tukey’s honestly significant difference, P < 0.05). Quantitative reverse transcription PCR (qRT–PCR) analysis of IAA30 ( C ), MIR408 ( D ), miR408-5p ( E ) and miR408-3p ( F ) expression in rice with auxin treatment under different time. G IAA30p-GUS and MIR408p-GUS staining in 7-d-old rice plants with and without 4 h 10 μM IAA treatment. Bars = 1 cm. H The relative intensity of GUS before and after IAA treatment shown in ( F ). Error bars indicate SD (Student’s t -test, ** P < 0.01, *** P < 0.001). Source data underlying ( B – F , H ) are provided as a Source Data file. Full size image To experimentally test whether miR408-5p can regulate IAA30 and IAA19 , we performed a luciferase (LUC)-based reporter assay, in which IAA30 or IAA19 were transiently expressed in Nicotiana benthamiana leaves under the control of their own promoter in the presence of miR408-5p (Fig. 2B and S2B ). On the one hand, the LUC signal was suppressed when both the wild-type IAA30 3’UTR and miR408-5p were introduced simultaneously, while it remained consistent when the mutated target sites of IAA30 and miR408-5p were co-expressed (Fig. 2B , Fig. S3A , B ). On the other hand, co-expression of IAA19 and miR408-5p did not result in a profound reduction of LUC intensity (Fig. S2B ). These results indicate that IAA30 rather than IAA19 is regulated by miR408-5p. Given the fact that the involvement of IAA proteins in auxin signaling is conserved among monocots and dicots [32] , we asked whether the targeting of IAA genes by miR408-5p is similarly conserved in different plants. To this end, we identified IAA orthologs in several representative monocots and dicots, and compared the sequence identities of their potential miR408-5p target sites, as well as other regions within IAA30s’ 3′UTRs (Fig. S4A ). We found the fragment of IAA30s that matches miR408-5p is more conserved in monocots than dicots (Fig. S4B ), implicating that the orthologues of IAA30s in monocots are more likely to be targeted by miR408-5p compared to those in dicots. Nonetheless, when we surveyed the complementarity of miR408-5p with IAA30 in six typical monocot species, we found that only IAA30s in rice and Aegilops tauschii showed potential targeting by miR408-5p (alignment score ≤ 4) (Fig. S4C ), indicating that the regulation of IAA30 by miR408-5p in monocots has not undergone a strong selection pressure during evolution. miR408-5p is induced by auxin in rice Since IAAs are involved in auxin signaling and miR408-5p targets IAA30 in rice, we wondered whether miR408-5p was responsive to auxin treatment. Consistent with the expression data of rice Aux/IAA members reported before [33] , our quantitative reverse transcription PCR (qRT–PCR) analysis showed that IAA30 was significantly induced in rice roots by 10 μM indole-3-acetic acid (IAA) application (Fig. 2C ). While the transcript of MIR408 was enhanced 4-fold after 4 h IAA treatment, the induction of miR408-5p examined by a stem-loop qPCR was milder than MIR408 , which was enhanced only 2-fold after 4 h IAA treatment and almost recovered after 8 h (Fig. 2D, E ). Moreover, we detected that the accumulation of miR408-3p was also enhanced by auxin treatment (Fig. 2F ). These results suggest that mature miR408-5p is subject to transcriptional and processing control in rice. To further determine the regulation of MIR408 and IAA30 by auxin, we generated transgenic rice plants expressing the GUS reporter gene driven by the MIR408 promoter ( MIR408p::GUS ) and IAA30 promoter ( IAA30p::GUS ), respectively, and analyzed their performance before and after IAA treatment. GUS staining showed that MIR408 was widely transcribed in rice plants, with particularly high expressions in roots, leaves, calli and leaf sheaths (Fig. S5 ). Moreover, we observed that the exogenous auxin treatment significantly enhanced the blue staining in both MIR408p::GUS and IAA30p::GUS transgenic plants (Fig. 2G, H ). These results revealed that the primary transcripts, mature small RNA as well as the target of miR408-5p in rice are induced by auxin application. Over-expression of miR408-5p in rice To gauge regulation of IAA30 by miR408-5p in vivo, we introduced MIR408 precursor under the UBIQUITIN ( UBI ) promoter into rice to generate MIR408 overexpression transgenic plants ( MIR408-OE ). A dramatic increase in miR408-3p and a decrease of its targets UCL7 and UCL8 indicated that the pri-miR408 was indeed constitutively expressed and correctly processed in transgenic plants (Fig. S6A ). As expected, the mature miR408-5p, as shown by stem-loop PCR, was significantly accumulated along with its precursor (Fig. S6B ). Since there was no developmental abnormality of roots existed in MIR408-OE plants compared with WT (Fig. S6C, D ), we planted MIR408-OE and WT on fluid nutrient medium for 3 days and then treated them with 10 μM IAA for 11 days to determine the biological significance of IAA30 by miR408-5p mediation. Unfortunately, we still could not find a noticeable difference between MIR408-OE and WT plants, although the status of primary roots and adventitious roots was easily observed to be altered by the application of exogenous auxin (Fig. S6E, F ). We were curious about why there was no morphological difference between MIR408-OE and WT plants after auxin treatment, because both miR408-5p and IAA30 were substantially induced by auxin. To address this question, we first generated loss-of-function of IAA30 mutants and observed their performances in rice (Fig. S7A ). Similar to MIR408-OE plants, iaa30 mutants lacked abnormal defects even when they were treated with auxin (Fig. S7B–E ). Given that there are 31 Aux/IAA genes in total in rice (Fig. S7F ) [33] , we speculated that the absence of root developmental differences between MIR408-OE and WT might be due to the redundancy of IAA30 with other IAAs. IAA11 was such a candidate according to its highest homology with IAA30 in rice (Fig. S7F ), and therefore we generated iaa30/iaa11 double mutants through the CRISPR-cas9 strategy (Fig. S7G ). Nevertheless, the plant root morphologies in iaa30/iaa11, MIR408-OE and WT were still similar even though all of them were grown under 10 μM IAA treatment (Fig. S7H–K ), implicating that not only IAA11 but also other IAAs may play redundant roles with IAA30 in auxin signaling in rice. miR408-5p is involved in auxin signaling Generally, IAA proteins play repressive roles in auxin signaling and may give rise to abnormal developments when they are over-accumulated in plants [34] . It has been shown that a gain-of-function mutation of IAA11 influences lateral root development and altered auxin signaling in rice [35] , we asked whether a similar performance would happen if IAA30 was overproduced. Therefore, we generated IAA30 overexpression lines ( IAA30-OE ) and strikingly found that they had longer primary roots and shorter crown roots than WT (Fig. S8A, B ), suggesting an important role of IAA30 in rice development, reminiscent that of IAA11 in rice [34] , [35] . To investigate the functional influence of miR408-5p on auxin signaling, we generated MIR408 knock-out mutants via CRISPR-cas9 approach (Fig. S8C ). Although no apparently developmental defects were observed under normal growth conditions (Fig. S8D, E ); the primary roots in mir408 mutants were significantly longer than those in WT when treated with 10 μM IAA (Fig. 3A, B ). Moreover, although there were no obvious changes in the number of adventitious roots in mir408 mutants compared with WT after IAA treatment, the three longest first-order adventitious roots in mir408 were much shorter than in WT, similar to those in IAA30-OE lines (Fig. 3A, D ). These results reflect that mir408 mutants are insensitive to auxin treatment compared to WT. Fig. 3: miR408-5p is involved in auxin signaling through regulation of IAA30. Representative photographs of 2-week-old mir408 ( A ), IAA30-OE ( C ), STTM-5p ( E ), mir408/iaa11/30 ( G ), STTM-5p/iaa11/30 ( I ) and respective WT plants under 10 μM IAA treatment. The red arrow indicates the primary root. Bar = 1 cm. B , D , F , H , J Primary root length, adventitious root number and the length of three longest first-order crown roots in 2-week-old WT and the indicated plants shown in ( A ), ( C ), ( E ), ( G ) and ( I ) under 10 μM IAA treatment. Error bars indicate SD (Multiple comparisons test, * P < 0.05; ** P < 0.01; *** P < 0.001; ns not significant; Tukey’s honestly significant difference, P < 0.05). Source data underlying ( B , D , F , H , J ) are provided as a Source Data file. Full size image Next, we attempted to determine the insensitivity of mir408 mutants to auxin is due to the loss of miR408-5p or miR408-3p activity. To this end, we made small tandem target mimic (STTM) constructs and introduced them into rice plants to compromise either miR408-5p or miR408-3p activity. The expression levels of miR408-3p and miR408-5p in the STTM-5p and STTM-3p transgenic plants, as detected by stem-loop qPCR, were found to be similar to those in WT, suggesting that blocking of miR408-5p and miR408-3p activity by STTM-5p and STTM-3p was specific (Fig. S9A, B ). Although there were no clear differences between STTM-5p and WT plants without an auxin treatment (Fig. S9C, D ), we observed an interesting phenomenon after the application of 10 μM IAA. STTM-5p exhibited longer primary roots and shorter adventitious roots compared to WT, which resembled the phenotype observed in mir408 mutants (Fig. 3E, F , and S9E–H ). In contrast, this phenotype was absent in STTM-3p plants (Fig. S10 ), suggesting that miR408-5p is more likely than miR408-3p to be involved in auxin signaling in rice. To further illustrate the involvement of MIR408 in auxin signaling through miR408-5p -directed target regulation, we performed a transcriptomic analysis using WT, STTM-5p, STTM-3p and IAA30-OE plants with or without a 4 h 10 μM IAA treatment. In our RNA-seq dataset, the number of differentially expressed genes (DEGs) by auxin treatment was similar in WT and STTM-3p , higher than that in STTM-5p and IAA30-OE plants (Fig. S11A–E , Supplementary Data 1 ). Furthermore, the functional categories of DEGs in STTM-5p and IAA30-OE were more similar to each other, distinct from those in WT and STTM-3p (Fig. S11F, G and Supplementary Data 2 ), providing further evidences that MIR408 regulates IAA30 predominately through miR408-5p. Finally, we determined the role of miR408-5p in auxin signaling dependent on IAA30 via genetics. When we introduced mir408 into iaa11/30 background through crossing, we found the insensitivity to auxin treatment in mir408 mutants was largely compromised (Fig. 3G, H , Fig. S12A, B ). Simultaneously, we transformed iaa11/30 mutants with STTM-5p constructs and obtained STTM-5p/iaa11/30 transgenic plants. Root phenotypic observation showed that the long primary roots observed in STTM-5p plants after IAA treatment disappeared when they were in the iaa11/30 background (Fig. 3I, J , Fig. S12C, D ), suggesting that IAA30 is genetically required for miR408-5p activity in auxin pathway. Collectively, these data reveal that miR408-5p mediates auxin signaling transduction in rice through regulating IAA30 . The regulatory machinery of IAA30 by miR408-5p It has been generally considered that the regulation of target by miRNA in plants is predominantly through mRNA cleavage [36] . miR408-5p seems to be analogous in this case, since overexpression of miR408-5p led to a decrease in IAA30 transcripts (Fig. 4A ). Fig. 4: Regulation manners of miR408-5p to IAA30 in rice . A Expressions of IAA30 in MIR408-OE , mir408 and STTM-5p plants. Error bars indicate SD (Multiple comparisons test, ** P < 0.01; *** P < 0.001; ns, not significant). Cleavage events of miR408-5p to IAA30 mRNA shown by degradome sequencing data obtained from MIR408-OE transgenic plants ( B ), explants from major root under 3d 10 μM 2,4-D treatment ( D ) and 14d rice callus induced by mature embryos ( E ). The red vertical bar indicates the positions of reads with the highest frequency mapped to the miR408-5p binding site. The green horizontal bar denotes miR408-5p targeting region. C Base pairing and the highest cleavage frequency of IAA30 3’UTR by miR408-5p observed in the indicated experiments shown in ( B ), ( D ), ( E ). The frequency of the sequenced 5′ends is plotted against the position in the IAA30 target site. F The constructs that were introduced into rice protoplast to determine the effect of miR408-5p on IAA30 . HptII , Hygromycin phosphotransferase II . RNA and protein abundance of IAA30 when normal IAA30 3’UTR (I) or mutated IAA30 3’UTR ( mUTR ) (II) construct shown in ( F ) was introduced into the protoplast from MIR408-OE ( G ), mir408 ( H ), STTM-5p ( I ) and STTM-3p ( J ) plants. The relative transcript and protein level of IAA30 were calculated using Actin as an endogenous control and were set to 1 in WT protoplast transformed with normal IAA30 3’UTR . RT- HptII was used to show the efficiency of plasmid transiently introduced into the indicated protoplast. Two independent transgenic lines were used to make protoplast. RT indicates transcript abundance determined by reverse transcription PCR; Anti denotes protein level examined by Western blot analysis using the indicated antibody. The number below each lane represents the relative amount compared with that in WT protoplast transformed with normal IAA30 3’UTR . K The constructs used to generate transgenic rice that was introduced Flag-tagged IAA30 with WT 3′UTR ( IAA30 ) or mutated 3′UTR ( IAA30m ) under control of the IAA30 native promoter. The red arrows with letter P mark the RT-PCR region for RNA determination. L RNA and protein abundance of IAA30 in WT and transgenic plants with indicated constructs shown in ( K ). The number below the lane represents the relative amounts of transcripts and proteins. M Representative photograph of 2-week-old WT, IAA30 and IAA30m transgenic plants under 10 μM IAA treatment. The red arrow indicates the primary root. Bar = 1 cm. N Primary root length, adventitious root number and the length of three longest first-order crown roots in 2-week-old WT, IAA30 and IAA30m transgenic plants under 10 μM IAA treatment. The different letters on top of each bar denote significant differences (Tukey’s honestly significant difference, P < 0.05). Source data underlying ( A , G – J , L , N ) are provided as a Source Data file. Full size image However, when we determined IAA30 expression by qRT-PCR in mir408 mutants, we were unable to detect any increase in IAA30 mRNA compared with that in WT (Fig. 4A ), although we readily detected an enhanced expression of UCL7 and UCL8 , two well-known targets of miR408-3p (Fig. S13A ). Furthermore, compared to WT, we did not observe an increase in IAA30 transcripts in STTM-5p plants (Fig. 4A ), whereas a conspicuous increase in the expression of UCL7 and UCL8 was detected in STTM-3p lines (Fig. S13B ), implying that the regulatory manner of miR408-5p on its target may differ from that of miR408-3p. Additionally, the expression of IAA30 is comparable in WT and STTM-3p plants (Fig. S13C ), indicating that miR408-3p may not be involved in IAA30 regulation in rice. When we conducted a 5′rapid amplification of complementary DNA (cDNA) ends (5′RACE) analysis to determine cleavage sites of IAA30 mRNA by miR408-5p, we were unable to detect any cleavage events on IAA30 mRNA. Moreover, despite the effectiveness of rice degradome databases in identification of rice mRNA targets, we did not detect any noteworthy cleavage events in the complementary region between miR408-5p and IAA30 (Fig. S13D ). These results indicated a non-canonical mode of action for miR408-5p in target regulation. The reduction of IAA30 expression in MIR408-OE plants coupled with the absence of enhanced IAA30 mRNAs in mir408 and STTM-5p plants led us to speculate that miR408-5p may change regulatory mechanism of IAA30 when its abundance is altered. To test this possibility, we first performed a degradome sequencing to examine IAA30 slicing events in MIR408-OE plants. Strikingly, IAA30 was cleaved by miR408-5p in the base-pairing region, although the major transcript ends deviated approximately 1 nucleotide upstream of the conventional cleavage site (between 9th and 10th relative to the 5′end of miRNA) (Fig. 4B, C ). 5′RACE experiment confirmed this cleavage event in MIR408-OE transgenic plants (Fig. S14A ). Additionally, a similar cleavage event was also detected in another degradome library from rice explants induced from major roots by a synthetic auxin, 2,4-dichlorophenoxyacetic acid (2,4-D) (Fig. 4C, D ). In addition, as miR408-5p is more abundant in rice callus than other tissues (Figs. S1B , S5 ), we constructed the third degradome library from 14-day-old rice callus that was generated from mature embryos under high auxin conditions. 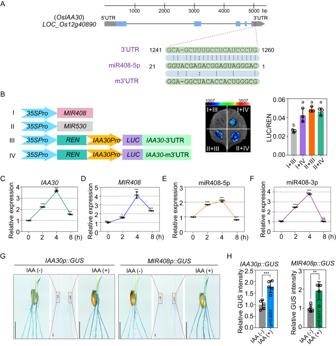Fig. 2: miR408-5p targetsIAA30and is induced by auxin in rice. AGene structure ofIAA30and alignments of miR408-5p with target sites inIAA303′UTR and mutant 3′UTR (m3′UTR).BValidation ofIAA30as miR408-5p target through transient expression analysis inN. benthamianaleaves. Left: The constructs inA. tumefacienstransiently introduced inN. benthamianaleaves. Middle: Representative photograph of firefly luciferase fluorescence signals when the indicated construct combinations were introduced inN. benthamianaleaves. Right: Relative reporter activity inN. benthamianaleaves expressing the indicated construct combinations. Error bars indicate SD (Tukey’s honestly significant difference,P< 0.05). Quantitative reverse transcription PCR (qRT–PCR) analysis ofIAA30(C),MIR408(D), miR408-5p (E) and miR408-3p (F) expression in rice with auxin treatment under different time.GIAA30p-GUSandMIR408p-GUSstaining in 7-d-old rice plants with and without 4 h 10 μM IAA treatment. Bars = 1 cm.HThe relative intensity of GUS before and after IAA treatment shown in (F). Error bars indicate SD (Student’st-test, **P< 0.01, ***P< 0.001). Source data underlying (B–F,H) are provided as a Source Data file. Interestingly, a consistent cleavage site of IAA30 was detected between the 8th and 9th nucleotide of miR408-5p, similar to that observed in MIR408-OE plants (Fig. 4C, E ). 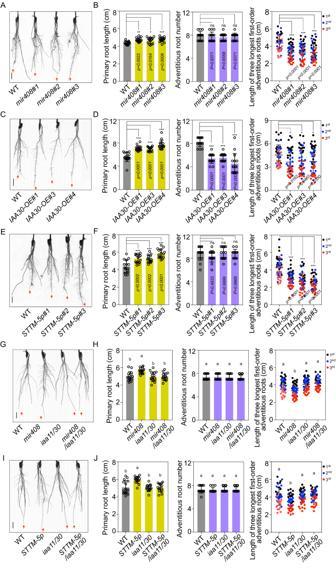Fig. 3: miR408-5p is involved in auxin signaling through regulation ofIAA30. Representative photographs of 2-week-oldmir408(A),IAA30-OE(C),STTM-5p(E),mir408/iaa11/30(G),STTM-5p/iaa11/30(I) and respective WT plants under 10 μM IAA treatment. The red arrow indicates the primary root. Bar = 1 cm.B,D,F,H,JPrimary root length, adventitious root number and the length of three longest first-order crown roots in 2-week-old WT and the indicated plants shown in (A), (C), (E), (G) and (I) under 10 μM IAA treatment. Error bars indicate SD (Multiple comparisons test, *P< 0.05; **P< 0.01; ***P< 0.001; ns not significant; Tukey’s honestly significant difference,P< 0.05). Source data underlying (B,D,F,H,J) are provided as a Source Data file. Together, these results suggest that miR408-5p down-regulates IAA30 by mRNA cleavage when it is artificially over-generated or accumulates above a basal threshold under high-auxin environments. Considering the difficulty in obtaining a specific antibody of IAA protein due to the high similarity of amino acids among different family members, we introduced a Flag-tagged IAA30 with WT 3′UTR (35S-Flag-IAA30-UTR) or mutated 3′UTR (35S-Flag-IAA30-mUTR) into rice protoplast to determine the protein accumulation in miR408-5p gain- and loss-of-function plants (Fig. 4F ). As anticipated, both the transcripts and proteins of IAA30 were reduced in MIR408-OE rice protoplasts (Fig. 4G , Fig. S14B ). However, the protein abundances but not the mRNA levels of IAA30 were increased in the protoplasts of mir408 mutants (Fig. 4H , Fig. S14B ). Furthermore, this increase in IAA30 protein was no longer observed when we introduced a mutated target site into IAA30 (Fig. 4H , Fig. S14B ). Next, we transiently expressed Flag-IAA30 in STTM-5p line protoplasts, and found that the protein, but not the mRNA, of IAA30 was higher in STTM-5p than in WT protoplasts (Fig. 4I , Fig. S14B ). By contrast, when we introduced 35S-Flag-IAA30-mUTR, the protein was accumulated similarly in protoplasts from WT and STTM-5p lines (Fig. 4I , Fig. S14B ). Moreover, when we used STTM-3p plants to generate protoplasts and introduced the same constructs, we found that neither mRNA nor protein of IAA30 was significantly enhanced in STTM-3p protoplasts compared with WT (Fig. 4J , Fig. S14B ). These results suggest that the translation of IAA30 is specially reinforced when miR408-5p activity is compromised. To further demonstrate the protein inhibition as the regulatory manner of IAA30 by miR408-5p under normal conditions, we generated transgenic rice expressing Flag-tagged IAA30 with either the WT 3′UTR or a mutated 3′UTR driven by the native IAA30 promoter (named IAA30 and IAA30m lines, respectively) (Fig. 4K ). Compared with IAA30 lines, although the mRNA levels were detected similarly, the protein of Flag-IAA30 was significantly higher in the IAA30m lines (Fig. 4L ), which result in longer primary roots and shorter adventitious roots, especially under the conditions with auxin treatment (Fig. 4M, N , Fig. S15A, B ). Taken together, our finding shows that miR408-5p mediates the regulation of IAA30 through translation repression under normal conditions, but switches to an mRNA digestion fashion if it is overproduced or enhanced by auxin. miR408-5p is regulated by miR156 and IPA1 in auxin signaling In Arabidopsis thaliana , miR408 is positively modulated by an SPL family protein, SPL7, to mediate the metabolism and development in response to copper and light [37] . We asked whether the precursor and mature miR408-5p could be regulated by SPL proteins in auxin pathway in rice. To this end, we first searched for GTAC-motifs, the potential binding elements of SPLs, in 1.5 kb promoter upstream of rice MIR408 . Like in A. thaliana , there were several GTAC-motifs in the MIR408 promoter, especially enriched within the 600 bp proximal region (Fig. 5A ). In rice, the gene IPA1 , which encodes SPL14, is a key regulator of architecture plasticity and has been considered as a new “Green Revolution” gene [20] , [23] . We examined the published chromatin immunoprecipitation (ChIP)-seq dataset of IPA1 [38] , and found a significant enrichment of IPA1 at MIR408 promoter, particularly in the proximal region (Fig. 5A ), suggesting that MIR408 is an authentic target of IPA1 and works downstream of IPA1 in the regulatory pathway. Yeast One-Hybrid (Y1H) analysis and ChIP-qPCR validated IPA1 as a plausible upstream regulator of MIR408 through interacting with its promoter proximal fragments (Fig. 5B, C ). Fig. 5: IPA1 regulated by miR156 acts upstream of miR408-5p in auxin signaling. A The association of IPA1 with MIR408 cis -elements in IPA1 ChIP-Seq datasets from three different rice tissues. The black bar on the promoter of MIR408 shown in the picture represents GTAC-motifs. P1 to P4 marked in red color denotes the fragments that were used to construct vectors for Yeast One-Hybrid (Y1H) analysis and a to d marked by blue color denotes the fragments that were examined by ChIP-qPCR. B Y1H analysis for the interaction of IPA1 with MIR408 promoter. Yeast cells growing on selective media without Leu and with the indicated concentration of Aureobasidin A (AbA) represent positive interactions. C ChIP-qPCR determination of IPA1 and MIR408 promoter interactions. GFP antibody was used for immunoprecipitation and Actin was used as an endogenous control to calculate the relative enrichment of IPA1 to different fragments of MIR408 promoter. D The reporter and effector constructs used for transient expression in N. benthamiana leaves for analysis of IPA1 activity to MIR408 activation. E Examination of IPA1 inductive activity to MIR408 transcription in N. benthamiana leaves. Left: Representative photograph of firefly luciferase fluorescence signals when the indicated constructs were introduced in N. benthamiana leaves. Right: Relative luciferase fluorescence signals in N. benthamiana leaves expressing the indicated reporters and effectors. Error bars indicate SD (Student’s t -test, ** P < 0.01). F qRT-PCR analysis of MIR408 and mature miR408-5p expressions in WT, MIR156-OE , IPA-OE and ipa1 rice plants. Error bars represent SD for three replicates. G Mature miR156 and IPA1 expressions in rice under 10 μM IAA treatment with the indicated time. H Representative phenotype of seedling roots of 2-week-old WT (ZH11), MIR156-OE transgenic plants and ipa1 mutants under 10 μM IAA treatment. The red arrow indicates primary roots. Bar = 1 cm. I Primary root length, adventitious root number and the length of three longest first-order crown roots in 2-week-old WT (ZH11), ipa1 mutants and MIR156-OE transgenic plants under 10 μM IAA treatment. Error bars indicate SD (Multiple comparisons test, ** P < 0.01; *** P < 0.001; ns, not significant). J Representative phenotype of seedling roots of 2-week-old WT (ZH11), MIR156-OE, MIR408-OE / MIR156-OE , MIR408-OE and NIP plants under 10 μM IAA treatment. The red arrow indicates primary roots. Bar = 1 cm. K Primary root length, adventitious root number and the length of three longest first-order crown roots in 2-week-old WT (ZH11), MIR156-OE, MIR408-OE / MIR156-OE , MIR408-OE and NIP plants under 10 μM IAA treatment. Error bars indicate SD (Tukey’s honestly significant difference, P < 0.05). L Representative phenotype of seedling roots of 2-week-old WT (ZH11), ipa1, MIR408-OE / ipa1 and a negative plant used for crossing without MIR408-OE (CK/ ipa1 ) under 10 μM IAA treatment. The red arrow indicates primary roots. Bar = 1 cm. M Primary root length, adventitious root number and the length of three longest first-order crown roots in 2-week-old WT (ZH11), ipa1, MIR408-OE / ipa1 and CK/ ipa1 plants under 10 μM IAA treatment. Error bars indicate SD (Tukey’s honestly significant difference, P < 0.05). Source data underlying ( C , E – G , I , K , M ) are provided as a Source Data file. Full size image To further confirm the effect of IPA1 on MIR408 expression, we made 35S::GUS and 35S::IPA1 effector constructs, and co-infiltrated them into N. benthamiana leaf epidermal cells along with a reporter system consisting of MIR408 promoter-driven LUC ( MIR408p::LUC ) and REN (Fig. 5D ). As shown in Fig. 5E , co-expression of MIR408p::LUC with IPA1 robustly enhanced the LUC activity, indicating that IPA1 positively regulates MIR408 . To trace the function of IPA1 to MIR408 in planta , we checked the expression of precursor and mature miR408-5p in IPA1 over-expression ( IPA1-OE ) and loss-of-function rice plants. As shown in Fig. 5F , MIR408 gene as well as miR408-5p were highly accumulated in IPA1-OE , while dramatically suppressed in ipa1 mutants and miR156 overproducing lines, in which IPA1 was silenced [39] . Since further expression analysis showed that mature miR156 was repressed whereas IPA1 was induced by IAA treatment (Fig. 5G ), we next gauged whether MIR156-OE plants and ipa1 mutants displayed insensitivity to auxin application. Compared with WT, both ipa1 mutant and MIR156-OE plants exhibited long seminal roots and short crown roots, similar to those in mir408 mutants and STTM-5p plants (Fig. 5H, I ). These results suggest that miR156 may inhibit the activity of miR408-5p in mediating auxin signaling through targeting IPA1 . It is worth noting that the number of adventitious roots under IAA treatment was lower in MIR156-OE , but comparable in ipa1 , mir408 and STTM-5p plants (Fig. 5I ), suggesting the decrease in adventitious root number caused by miR156 over-accumulation may be dependent on repression of other SPLs rather than IPA1 and miR408-5p. To determine the genetic relationship between MIR408 and MIR156 , we introduced MIR408-OE constructs into MIR156-OE plants by transformation, and noticed that the long primary roots and short adventitious roots in MIR156-OE compared to WT was partially restored when MIR408 was overexpressed (Fig. 5J, K ). Meanwhile, when we crossed ipa1 mutants with MIR408-OE plants, we found that the long seminal roots and short crown roots in ipa1 were significantly attenuated when MIR408-OE was introduced (Fig. 5L, M ). These data together indicate a genetic epistasis of miR408-5p to miR156 and IPA1 in rice auxin signaling. Overall, these results characterize a regulatory cascade in rice auxin signaling that is constituted by miR156- IPA1 -miR408-5p- IAA30 . miR156- IPA1 -miR408-5p- IAA30 circuit regulates leaf inclination in rice As we have demonstrated the regulation of IAA30 by miR408-5p in auxin signaling, we subsequently wondered about the biological significance of this module in rice. Leaf angle is an important agronomic trait of crops that influences photosynthetic efficiency and yield [40] . Several studies have implicated the significance of auxin in regulation of leaf inclination [41] , [42] , [43] . In our IAA30-OE transgenic lines, we found an enlarged leaf inclination compared with WT (Fig. S16A–C ). The paraffin section revealed that the cell width of the fourth layer parenchyma cells at the adaxial side of the lamina joint of flag leaves was significantly increased in IAA30-OE compared to WT (Fig. S16D, E ), consistent with the previous report that auxin-mediated leaf inclination regulation predominantly depends on the change of cell size rather than cell number [41] . By phenotypic observation, we found that both mir408 mutants and STTM-5p plants showed increased leaf angles after heading (Fig. 6A–F ), although there was no obvious reduction of leaf inclination in our MIR408-OE plants (Fig. S16F–J ). Most flag leaves on major stems with panicles in mir408 mutants and STTM-5p plants were above 60°, in contrast with those below 30° in WT (Fig. 6B, E ). When we calculated the ratio of inclination of leaves≥90° in all stems harboring panicles, we observed that flag leaves over 30% in mir408 mutants and 20% in STTM-5p plants were more than 90°, while this ratio was below 5% in WT (Fig. 6C , F ). Meanwhile, we did not observe a distinctive difference in leaf angles between STTM-3p and WT plants (Fig. 6G– I ). In line with these phenotypic observations, the longitudinal sections displayed an increased cell width of the adaxial side of lamina joint in mir408 mutants and STTM-5p plants, while no alteration was found in WT and STTM-3p lines (Fig. 6J, K ). Thus, the presence and the absence of enlarged leaf inclination in STTM-5p and STTM-3p plants, respectively, defined that regulation of leaf inclination by MIR408 is mainly through miR408-5p. Fig. 6: miR156- IPA1 -miR408-5p- IAA30 circuit regulates rice leaf inclination. Phenotypic observations of mir408 ( A ), STTM-5p ( D ) and STTM-3p ( G ) and respective WT plants (Bars = 10 cm). Boxed regions are enlarged to the performance of flag leaves with panicles (Bars = 1 cm). White arrows indicate the lamina joints. Inclination of flag leaves on the main stem with panicles in mir408 ( B ), STTM-5p ( E ) and STTM-3p ( H ) and respective WT plants. Angles of flag leaf at 40 days after heading were measured and data are presented as means ± SD (standard deviation, n = 12). Statistical analysis was conducted by using Multiple comparisons test (*** P < 0.001; ns not significant). The ratio of flag leaves with angle≥90°from all flag leaves on stems with panicles in mir408 ( C ), STTM-5p ( F ) and STTM-3p ( I ) and respective WT plants. Statistical analysis was executed by using Multiple comparisons test (*** P < 0.001; ns not significant). J Longitudinal section of the adaxial region of the lamina joint in WT, mir408 , STTM-5p and STTM-3p flag leaves at 40 days after heading. The marked regions in red color were magnified to highlight the differences. K Cell length and cell width of adaxial parenchyma cells of lamina joint in WT, mir408 , STTM-5p and STTM-3p plants. The fourth layer parenchyma cells at the adaxial side were calculated and statistically analyzed by Multiple comparisons test (*** P < 0.001; ns not significant). L Typical plant phenotypes of WT (ZH11), miR156-OE transgenic plants and ipa1 mutants (Bars = 10 cm). Boxed regions are enlarged to the performance of flag leaves with panicles (Bars = 1 cm). White arrows indicate the lamina joints. M Inclination of flag leaf on the main stem with panicle in WT (ZH11), miR156-OE and ipa1 plants. N The ratio of flag leaves with angle≥90°from all flag leaves on stems with panicles in WT (ZH11), miR156-OE and ipa1 plants. O Longitudinal section of the adaxial region of the lamina joint in WT (ZH11), miR156-OE and ipa1 flag leaves at 40 days after heading. P Cell length and cell width of adaxial parenchyma cells of lamina joint in WT (ZH11), miR156-OE and ipa1 plants. Phenotypic comparisons in WT (ZH11), miR156-OE, miR408-OE/miR156-OE , miR408-OE , NIP plants ( Q ) and in WT (ZH11), ipa1, MIR408-OE / ipa1 and CK/ ipa1 plants ( T ). Inclination of flag leaf on the main stem with panicle in WT (ZH11), miR156-OE, miR408-OE/miR156-OE , miR408-OE , NIP plants ( R ) and in WT (ZH11), ipa1, MIR408-OE / ipa1 and CK/ ipa1 plants ( U ). The ratio of flag leaves with angle ≥90° from all flag leaves on stems with panicles in WT (ZH11), miR156-OE, miR408-OE/miR156-OE , miR408-OE , NIP plants ( S ) and in WT (ZH11), ipa1, MIR408-OE / ipa1 and CK/ ipa1 plants ( V ). Source data underlying ( B , C , E , F , H , I , K , M , N , P , R , S , U and V ) are provided as a Source Data file. Full size image Additionally, compared with WT, very few leaves in IAA30 plants were observed that enhanced their angles, while those were readily found in IAA30m lines (Fig. S16K–M ), further indicating that the miR408-5p-IAA30 regulon mediates leaf development in rice. We could not observe a visible change in leaf angle in MIR408-OE plants (Fig. S16F–J ), possibly because only a decrease of IAA30 cannot affect leaf inclination due to the heavy redundancy of IAA family proteins. Because IPA1 promotes miR408-5p accumulation through associating with MIR408 cis-elements, IPA1 likely represses leaf inclination. Indeed, we found that the flag leaf angles in miR156-OE plants and ipa1 mutants, in which miR408-5p accumulations were decreased, were almost 100°, much higher than that of WT (Fig. 6L–N ). Moreover, cytological analysis showed that the width of the fourth layer cells of the lamina joint at adaxial side was substantially increased in miR156-OE and ipa1 compared to WT (Fig. 6O, P ), further implicating their enlarged leaf inclinations possible because of the miR408-5p deficiency. In addition, the enlarged leaf inclination in miR156-OE and ipa1 was remarkably compromised when overexpression of MIR408 was introduced, indicating that regulation of leaf angle development by miR156 and IPA1 in rice is genetically dependent on the potential role of miR408-5p (Fig. 6Q–V ). Taken together, our data illustrate the biological significance of the modulatory circuit formed by miR156- IPA1 -miR408-5p- IAA30 in auxin signaling in rice. The effects of miR393- TIR1/AFB module on miR156- IPA1 -miR408-5p- IAA30 circuit in rice Because auxin signaling primarily begins with the sensing of auxin molecules by TIR1/AFBs F-box receptor proteins, we pursued whether the response of miR408-5p to auxin was also dependent on these receptors. For this purpose, we examined the expression of MIR408 and miR408-5p accumulations in two miR393 overexpression rice lines ( MIR393a-OE and MIR393b-OE ), in which major TIR1/AFBs genes were silenced [44] . Intriguingly, we observed that both MIR408 and miR408-5p showed reduced responsiveness to IAA application in miR393 overproducers compared to WT (Fig. S17A, B ), which is consistent with the results obtained from tir1 mutants (Fig. S17C, D ). These data collectively show that auxin receptors are essential for the induction of miR408-5p by auxin. In accordance with this, we also observed a greater bending of the lamina joint in miR393a-OE plants (Fig. S18A–E ), similar to those in mir408 and STTM-5p . Next, we investigated whether miR393-TIR1/AFBs module influenced the expressions of miR156 and IPA1 , the upstream regulators of miR408-5p. We found that both the basal expression and induction of IPA1 by auxin were dramatically compromised in MIR393a-OE and MIR393b-OE plants (Fig. S19A ), suggesting that auxin reception by TIR1/AFBs is important for IPA1 regulation. However, when we measured the abundance of mature miR156 in MIR393a-OE and MIR393b-OE plants, we found no difference before auxin treatment compared with WT (Fig. S19B ). Nonetheless, when we detected the repression of miR156 after auxin treatment, we found it was significantly enhanced by overexpression of miR393 (Fig. S19B ), indicating that the response to high auxin environment, but not the basal expression of miR156 in rice, is affected by the miR393-TIR1/AFBs module. Here, we present a regulatory network in rice involving three miRNAs that mediates plant architecture through auxin signaling (Fig. 7 ). Most surprisingly, we find that miR408-5p controls IAA30 through translational repression under normal conditions, while shifts to mRNA degradation to silence it when miR408-5p is induced by high auxin perception. To our knowledge, this is the first study that clearly elucidate the circumstance under which miRNA can switch regulatory modes in target regulation. Fig. 7: Working model of auxin signaling involving miR408-5p regulation in rice. Compared with that in low auxin environment, rice in high auxin condition represses miR156 and promotes more association of IPA1 with MIR408 cis-element to trigger higher accumulations of mature miR408-5p, thereby leading to switch miR408-5p action from translation repression to mRNA cleavage. In addition to a higher contribution from canonical receptor-mediated auxin signaling, more robust regulation of IAA30 by miR408-5p in rice through mRNA cleavage results in an enhanced auxin response in a high than in a low auxin environment. Full size image miRNA-miRNA interaction as a master regulatory circuit in plant development Indeed, the versatile roles of miRNA-target modules in plants are being gradually uncovered. The verified targets of plant miRNAs encompass a diverse range of modulatory proteins, especially transcription factors. This implies that miRNA-mediated targets may constitute a regulatory circuit through modulating another miRNA and its targets, allowing for hierarchical and efficient participation in plant development or adaptation. For example, miR156 represses miR172 through suppressing SPL3 , which to release a class of APETALA 2 transcription factors that control growth transition and reproductive development [45] . In leaf morphogenesis, miR164 targets CUP-SHAPED COTYLEDON 2 mRNA, which is decoyed by miR319-TEOSINTE BRANCHED 3, a key regulon involved in a gradual increase of leaf complexity in the newly formed organs [46] . Due to the high conservation of these miRNAs and targets among diverse plants, such regulatory cascades are vital in plant growth and have undergone strong selective pressure during evolution. We find herein that IPA1, an important contributor to the desirable architecture trait in rice, promotes miR408-5p accumulation through binding MIR408 cis -elements. As miR156 and miR393 regulate IPA1 , the hierarchy interaction between these miRNAs is critical to regulate leaf lamina joint development in rice. Interestingly, the repression of miR156 by exogenous auxin treatment is exacerbated rather than attenuated when the canonical auxin receptors TIR1/AFBs are inhibited, implicating that regulation of miR156 by auxin may rely on alternative auxin receptors, such as Auxin-binding protein 1 (ABP1) as illustrated recently [47] , or be subject to feed-back regulations by other components in the auxin signaling pathway. Contribution of translation repression and mRNA decay in silencing target by a miRNA During the last two decades, numerous studies revealed two modes of negative regulation by miRNA on targets: translation repression and mRNA cleavage. The degree of complementarity between the miRNA and its target has been generally considered as a key determinant of the mechanism used, such that perfect match facilitates cleavage, while less pairing promotes to suppress protein translation [8] . In animals, most miRNAs display less matches to their target mRNAs than in plants, so translation inhibition is considered as the critical activity of miRNAs in animals, preceding target mRNA decay [14] . Unlike animal miRNA, plant miRNA matches nicely with targets, and thereby often presents as a guide for target RNA cleavage. Another interpretation of limited events of translation inhibition in plants is that plants lack GW182 homolog proteins, which are the core components for miRNA-mediated translational repression in animals [14] . However, several conserved miRNAs, including miR156, miR172, miR398, miR164 and miR165/166, have been reported that translation repression is engaged in target silencing, independent of slicing the same gene transcripts [3] , [5] , [6] , [10] . Despite a deficiency in miRNA-mediated translational inhibition, several mutants in plants, such as katanin1 ( knt1 ) and suo1 , display only mild abnormality in development, whereas others, including ago1-27, altered meristem program 1 ( amp1 ) and like-amp1 ( lamp1 ), exhibit severe pleiotropic growth defects [8] , [10] , [12] . Thus, it is difficult to conclude whether translation repression by miRNA is also a fundamental approach to target regulation as mRNA cleavage in plants. If the two silencing modes coexist and cannot be separated, the physiological importance of each mode in miRNA action remains unresolved. In the present study, we uncover that miR408-5p in rice represses target protein translation under the ordinary circumstance, but it switches mRNA degradation, thereby enhancing regulatory efficiency when plants sense an auxin signal. Our finding separates the two mechanisms of miRNA actions temporally and demonstrates their balance is essential for rice architecture plasticity, such as leaf inclination. To date, there have been very few reports on the functions of non-conserved miRNAs in plants, mainly due to their low abundances compared to the conserved miRNAs. Nevertheless, miR834, an Arabidopsis -specific miRNA, that has received more attention because it silences CIP4 by translation repression [8] . Since miR834 is a non-conserved miRNA and almost perfectly matches with the target, it has been proposed that young miRNA may be predominately utilize the translational repression pathway regardless of the mismatches in small RNA-target hybrids [8] . This prospective appears reasonable, because miR408-5p, which regulates IAA30 in rice, performs translational control of IAA30 under normal environments. Nonetheless, miR408-5p can switch action modes to mRNA cleavage for IAA30 regulation when subject to a high auxin signal. Considering that miR408-5p is present and targets IAA30 orthologs in a few monocots, we propose that miRNAs with intermediate conservation in plants generally mediate the inhibition of target protein translation, while they may promptly change their mode of action to mRNA clearance, thereby enhancing target regulation efficiency under specific conditions. It is noteworthy that miR408-3p is one of the most ancient miRNAs in land plants [48] . A couple of studies have shown that miR408-3p is involved in multiple physiological processes across diverse plants, including photosynthesis, fertility, biomass and tolerance against adverse environments through efficient suppression of conserved target expressions [25] , [26] , [49] , [50] , [51] , [52] . In the present study, we discover that miR408-5p, another mature miRNA generated from the same precursor in rice, mediates auxin signaling cascade and development. Therefore, considering the versatile roles of MIR408 in plants, it has a huge potential to serve as an integrator for crop improvement with multiplex desirable traits. Plant material and growth conditions Japonica rice ( Oryza sativa ) variety Nipponbare (NIP) was used for auxin treatment, as well as for cloning of MIR408 and IAA30 genes, plant transformation and protoplast isolation, unless otherwise specified. Rice seeds were germinated in sterilized water and planted in a growth chamber under a 14 h light (28 °C)/10 h dark (22 °C) cycle for the growth of transgenic plants. For auxin sensitivity assay in roots, rice seeds were surface-sterilized, and imbibed for 48 h in distilled water under dark condition at 30 °C. The synchronously germinated seeds were then grown on a fluid nutrient medium for 3 days and then supplemented with the indicated concentration of IAA for 11 days. The lengths of the primary and adventurous seedling roots of indicated lines were then measured and analyzed. For rice transformation, mature rice embryos were used and placed on N6 callus initiation medium supplemented 2.5 mg/L 2,4-D to induce callus. Rice plants for leaf angle determination and paraffin sections were grown in the paddy field with routine management in Changxing and Hangzhou in Zhejiang Province of China under natural summer field conditions. Three independent transgenic lines with a single copy of the insertions were used to observe the phenotypes unless otherwise specified. All transgenic plants analyzed in our study were T 3 generation homozygous plants. Plasmid construction The coding sequence of IAA30 was amplified from rice cDNA through PCR, and a 0.6 kb sequence containing MIR408 precursor from rice DNA was cloned into a modified pCAMBIA1390 with a maize UBI promoter for over-expression in rice. To create the STTM-3p and STTM-5p constructs, the sequences with KpnI and BamHI sites of STTM structure against miR408-3p and miR408-5p were produced by overlapping PCR, respectively. These sequences were then cloned into the modified pCAMBIA1390. The mir408 , iaa30 and iaa11/30 mutants in rice were generated by CRISPR-cas9 strategy. The sgRNA and constructs were designed and made essentially as described before [53] . For transient expression of IAA30 in rice protoplasts, IAA30 with its 3′UTR was amplified from NIP rice cDNA. Target site mutated IAA30 at 3′UTR (mUTR) was generated through overlapping PCR. Both Flag-tagged IAA30-UTR and Flag-tagged IAA30-mUTR were constructed with a CaMV35S promoter for transient overexpression in rice protoplasts. To construct 35S::MIR408-NOS , IAA30pro::LUC-IAA30-3’UTR , IAA30pro::LUC-IAA30 m3’UTRs, IAA19pro::LUC-IAA19-3’UTR and IAA19pro::LUC-IAA19 m3’UTR for infection of Nicotiana benthamiana , MIR408 , IAA30 3’UTR and IAA19 3’UTR were amplified from cDNA, while the promoter of IAA30 and IAA19 were amplified from DNA of rice plants. MIR408 was introduced into a modified pCAMBIA2300 under the control of CaMV35S promoter, while LUC-IAA30-3’UTR , LUC-IAA30-m3’UTRs , LUC-IAA19-3’UTR and LUC-IAA19 m3’UTR were inserted behind their respective 2 kb native promoter. For luciferase imaging assays, the coding region of IPA1 was obtained from NIP cDNA and inserted into pCAMBIA2300 under the control of CaMV35S promoter, while the promoter of MIR408 was constructed into the modified pGreen0800 II-LUC vector, which carries the Renilla ( REN ) gene for calculating the relative LUC activity. IAA30pro::LUC-IAA30-3’UTRs and IAA30pro::LUC-IAA30 m3’UTRs constructs were also transformed into rice to generate IAA30 and IAA30m plants, respectively. For the IAA30pro::GUS and MIR408pro::GUS construct, the CaMV35S promoter in pCAMBIA1301 was replaced by a 2.1 kb promoter before the start codon of IAA30 and a 2.9 kb promoter before the precursor of MIR408 , respectively. All binary expression vectors were introduced into Agrobacterium tumefaciens strain AGL1 for rice transformation and EHA105 for the infiltration of tobacco leaves. All primers used for plasmid construction are listed in Supplementary Data 3 . Transfection of rice protoplasts and western blots Generally, the plasmids 35S-Flag-IAA30-UTR or 35S-Flag-IAA30-mUTR were transformed into rice protoplast according to the protocols described before [54] . Briefly, Ten-day-old WT and indicated transgenic rice seedlings were used to isolate protoplasts. Around 200 μl protoplast suspension (containing ~2 × 10 5 protoplasts) was transfected with 10 μg of plasmid in a 110 μl PEG solution. The transformation mixture was incubated in dark for 15 min at 28˚C, then diluted with 1 ml W5 solution (NaCl, 154 mM; CaCl 2 , 125 mM; KCl, 5 mM; MES, 2 mM, pH 5.7) and centrifuged at 120 g for 3 min. Protoplasts were suspended in W1 solution (Mannitol, 0.5 M; KCl, 20 mM; MES, 4 mM, pH 5.7) and transferred into multi-well plates and incubated at 28 °C for 16 h. Total proteins were extracted from half of the transfected protoplasts, and the remaining protoplasts were used for RNA extraction and RT-PCR. For immunoblot analyses, total proteins were isolated from the corresponding protoplasts of WT and transgenic seedlings. The proteins were separated by sodium dodecyl sulfate-polyacrylamide gel electrophoresis, transferred to polyvinylidene difluoride membranes, immunoblotted with corresponding commercial antibodies, and detected using High-sig ECL Western Blotting Substrate (Tanon). Homology based identification of miR408-5p and IAA30 target sequences in diverse plants using BLAST Mature miRNAs and miRNA precursors for MIR408 in 14 selected plant species were retrieved from the miRBase database (version 22). The genomic sequences were downloaded from the Ensembl Plants database (version 50) except for citrus sinensis , which was downloaded from the Orange ( citrus sinensis ) genome annotation project (version 2.0) ( http://citrus.hzau.edu.cn/orange /download/index.php) [55] . The orthologous genes of IAA30 among species were identified based on reciprocal best blast hits (RBH) with BlastN (Query identity = 50% and e = 1 × 10 −10 ). Sequences of MIR408 precursors and IAA30 in the 14 selected plant species were aligned using MAFFT (version 7). The sequence alignment files were used to calculate the sequence identity at each position. An unrooted phylogenetic tree of MIR408 precursors was constructed using RAXML with the maximum-likelihood (ML) method. The expression matrix for the two mature miRNAs from MIR408 , MIR166a , MIR167a , MIR168a , MIR319a and MIR396e were retrieved from the PmiRExAt database ( http://pmirexat.nabi.res.in/datashow.html ) [30] . GUS staining Seedlings and plants of MIR408p-GUS and IAA30p-GUS transgenic rice were stained in a GUS staining solution (2 mM 5-bromo-4-chloro-3-indolyl-b-D-glucuronic acid, 50 mM NaH 2 PO 4 /Na 2 HPO 4 buffer, 2 mM each K 3 Fe(CN) 6 /K 4 Fe(CN) 6 , 10 mM Na 2 EDTA and 0.1% Triton X-100) and incubated at 37 °C for 8 to 12 h. After GUS staining, chlorophyll was removed using 70% ethanol. RT-PCR and real time qRT-PCR Total RNAs were isolated from rice roots using the Trizol reagent (Takara) unless otherwise specified. After determining the RNA quantification, the RNAs were reverse transcribed by M-MLV (Promega) by using oligo (dT). The cDNAs were then used as templates for direct PCR or quantitative PCR. Quantitative PCR was performed using SYBR Premix (Invitrogen) on StepOnePlus™ System (Thermo-Fisher) and the Actin gene was used as an endogenous control. The abundance of mature miRNA was determined by the stem-loop qRT-PCR as described before and U6 was used as an endogenous control. Three biological repeats of each qRT-PCR were conducted and each value indicates the average with the standard error. All primer sequences are listed in Supplementary Data 3 . Degradome sequencing and analysis Degradome libraries were prepared from rice with high miR408-5p accumulations using three different materials. The first material that we used to isolate total RNA was seedlings of MIR408-OE transgenic plants, the second material was explant using primary roots under 3d 10 μM 2,4-D treatment, and the third material was 14d callus induced from rice mature embryo on N 6 callus initiation medium with 2.5 mg/L 2,4-D application. Degradome library construction was performed with a slight modification as previously described [56] , [57] . Briefly, poly (A) enriched RNA was mixed and annealed using biotinylated random primers. RNAs with 5’-monophosphates were ligated to 5′adapters and the libraries were subject to single-end sequenced using the 5′adapter on an Illumina HiSeq 2500 (LC-Bio, China). The sequencing data were analyzed using CleaveLand3.0. The degradome reads were matched to generate the degradome density file using script “CleaveLand3_map2dd.pl”. Reads that mapped to the predicted IAA30 target sites were utilized to determine the positions of the 5′transcript ends using an in-house Perl script. A couple of sets publicly available of degradome sequencing data from wild-type seedlings (PRJNA118841, PRJNA123507, PRJNA120547, PRJNA263869, PRJNA170713, PRJNA263450, PRJNA596446, PRJNA627552, PRJNA594662, PRJNA630172, PRJNA561367, PRJNA486509, PRJNA480216, PRJNA388531, PRJNA182050, PRJNA277443 and PRJNA263869) were used as control samples of rice plants without auxin treatments [58] , [59] , [60] , [61] , [62] , [63] , [64] , [65] , [66] , [67] , [68] , [69] , [70] , [71] , [72] , [73] , [74] . Mapping of the IAA30 mRNA cleavage sites by 5′RACE For mapping the cleavage site in IAA30 mRNA, total RNA was isolated from MIR408-OE transgenic plants and poly(A) + mRNA was purified by Capture mRNA Kit (Qiagen, Germany). 5´ RACE was performed according to the instruction manual provided in the Kit of 5´ RACE System for Rapid Amplification of cDNA Ends (Invitrogen life science technologies, USA). PCR products were gel purified and cloned into pMD18-T vector (Takara, Japan) for sequencing. The oligo primers are listed in Supplementary Data 3 . Transcriptome sequencing and analysis Synchronously germinated seeds of STTM-5p , STTM-3p , IAA30-OE and WT rice were grown on a fluid nutrient medium for 3 days and treated with 10 μM IAA for RNA isolation. Transcriptome libraries were constructed for each root sample individually, and then sequenced using Hiseq 2500 (LC-Bio, Hangzhou, China). Three biological replicates were conducted for each treatment. The clean reads from each sample were aligned to rice reference genome (IRGSP-1.0) using HISAT2 software [75] . Only uniquely mapped reads were used for expression quantification with StringTie v2.0. Differential expression analysis for individual studies was performed using Ballgown package [76] . Gene expression was quantified as fragments per kb per million reads (FPKM). Genes with a fold-change greater than 2.0 and an adjusted p-value less than 0.05 were considered as differentially expressed genes (DEGs), which were subjected to GO functional enrichment analyses using AgriGO v2.0 [77] . ChIP-qPCR The wild-type rice and IPA1pro:: mIPA1-GFP transgenic plants obtained from Dr. Jiayang Li’s lab were used for ChIP assays according to the EpiQuikTM Plant ChIP Kit protocol (Epigentek, USA). Briefly, 2 g samples were crosslinked with 1% (v/v) formaldehyde under 10 min vacuum and then ground to powder in liquid nitrogen. 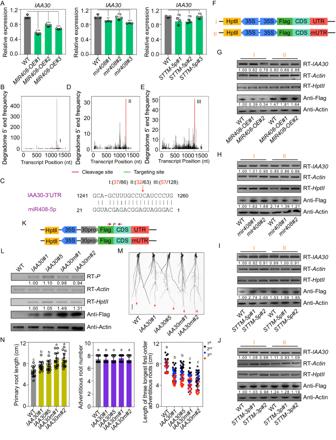Fig. 4: Regulation manners of miR408-5p toIAA30in rice. AExpressions ofIAA30inMIR408-OE,mir408andSTTM-5pplants. Error bars indicate SD (Multiple comparisons test, **P< 0.01; ***P< 0.001; ns, not significant). Cleavage events of miR408-5p toIAA30mRNA shown by degradome sequencing data obtained fromMIR408-OEtransgenic plants (B), explants from major root under 3d 10 μM 2,4-D treatment (D) and 14d rice callus induced by mature embryos (E). The red vertical bar indicates the positions of reads with the highest frequency mapped to the miR408-5p binding site. The green horizontal bar denotes miR408-5p targeting region.CBase pairing and the highest cleavage frequency ofIAA303’UTR by miR408-5p observed in the indicated experiments shown in (B), (D), (E). The frequency of the sequenced 5′ends is plotted against the position in theIAA30target site.FThe constructs that were introduced into rice protoplast to determine the effect of miR408-5p onIAA30.HptII,Hygromycin phosphotransferase II. RNA and protein abundance ofIAA30when normalIAA30 3’UTR(I) or mutatedIAA30 3’UTR(mUTR) (II) construct shown in (F) was introduced into the protoplast fromMIR408-OE(G),mir408(H),STTM-5p(I) andSTTM-3p(J) plants. The relative transcript and protein level ofIAA30were calculated usingActinas an endogenous control and were set to 1 in WT protoplast transformed with normalIAA30 3’UTR. RT-HptIIwas used to show the efficiency of plasmid transiently introduced into the indicated protoplast. Two independent transgenic lines were used to make protoplast. RT indicates transcript abundance determined by reverse transcription PCR; Anti denotes protein level examined by Western blot analysis using the indicated antibody. The number below each lane represents the relative amount compared with that in WT protoplast transformed with normalIAA30 3’UTR.KThe constructs used to generate transgenic rice that was introduced Flag-tagged IAA30 with WT 3′UTR (IAA30) or mutated 3′UTR (IAA30m) under control of theIAA30native promoter. The red arrows with letter P mark the RT-PCR region for RNA determination.LRNA and protein abundance ofIAA30in WT and transgenic plants with indicated constructs shown in (K). The number below the lane represents the relative amounts of transcripts and proteins.MRepresentative photograph of 2-week-old WT,IAA30andIAA30mtransgenic plants under 10 μM IAA treatment. The red arrow indicates the primary root. Bar = 1 cm.NPrimary root length, adventitious root number and the length of three longest first-order crown roots in 2-week-old WT,IAA30andIAA30mtransgenic plants under 10 μM IAA treatment. The different letters on top of each bar denote significant differences (Tukey’s honestly significant difference,P< 0.05). Source data underlying (A,G–J,L,N) are provided as a Source Data file. The nuclei and chromatin complexes were isolated, sonicated and then incubated with anti-GFP antibody for immunoprecipitation. The precipitated DNA was recovered and dissolved in water for qPCR with the indicated primers using SYBR Premix (Invitrogen) on StepOnePlus™ System (Thermo-Fisher). The fold enrichment was calculated between IPA1pro:: mIPA1-GFP and the WT input. Fold of enrichment in IPA1pro:: mIPA1-GFP against the WT was calculated from three independent qPCR. Luciferase imaging assays To determine the effects of miR408-5p on IAA30 and IAA19 , equal concentrations and volumes of A. tumefaciens strains EHA105 harboring indicated WT and mutated target site of IAA30 or IAA19 along with MIR408 or control constructs were co-infiltrated into N. benthamiana leaves. At least four leaves from independent N. benthamiana plants were infiltrated and observed the fluorescence signal. To detect inductive effects of IPA1 on MIR408 transcription, equal concentrations and volumes of A. tumefaciens strains EHA105 harboring ProMIR408::LUC construct with CaMV35S::IPA1 or control constructs were infiltrated into N. benthamiana leaves. For observation of the fluorescence signal, the injected tobacco leaves were kept in a dark condition for 5 min after a spray of Luciferin (100 μM). 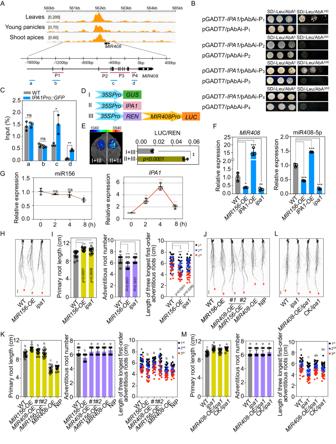Fig. 5: IPA1 regulated by miR156 acts upstream of miR408-5p in auxin signaling. AThe association of IPA1 withMIR408 cis-elements in IPA1 ChIP-Seq datasets from three different rice tissues. The black bar on the promoter ofMIR408shown in the picture represents GTAC-motifs. P1 to P4 marked in red color denotes the fragments that were used to construct vectors for Yeast One-Hybrid (Y1H) analysis and a to d marked by blue color denotes the fragments that were examined by ChIP-qPCR.BY1H analysis for the interaction of IPA1 withMIR408promoter. Yeast cells growing on selective media without Leu and with the indicated concentration of Aureobasidin A (AbA) represent positive interactions.CChIP-qPCR determination of IPA1 andMIR408promoter interactions. GFP antibody was used for immunoprecipitation andActinwas used as an endogenous control to calculate the relative enrichment of IPA1 to different fragments ofMIR408promoter.DThe reporter and effector constructs used for transient expression inN. benthamianaleaves for analysis of IPA1 activity toMIR408activation.EExamination of IPA1 inductive activity toMIR408transcription inN. benthamianaleaves. Left: Representative photograph of firefly luciferase fluorescence signals when the indicated constructs were introduced inN. benthamianaleaves. Right: Relative luciferase fluorescence signals inN. benthamianaleaves expressing the indicated reporters and effectors. Error bars indicate SD (Student’st-test, **P< 0.01).FqRT-PCR analysis ofMIR408and mature miR408-5p expressions in WT,MIR156-OE,IPA-OEandipa1rice plants. Error bars represent SD for three replicates.GMature miR156 andIPA1expressions in rice under 10 μM IAA treatment with the indicated time.HRepresentative phenotype of seedling roots of 2-week-old WT (ZH11),MIR156-OEtransgenic plants andipa1mutants under 10 μM IAA treatment. The red arrow indicates primary roots. Bar = 1 cm.IPrimary root length, adventitious root number and the length of three longest first-order crown roots in 2-week-old WT (ZH11),ipa1mutants andMIR156-OEtransgenic plants under 10 μM IAA treatment. Error bars indicate SD (Multiple comparisons test, **P< 0.01; ***P< 0.001; ns, not significant).JRepresentative phenotype of seedling roots of 2-week-old WT (ZH11),MIR156-OE, MIR408-OE/MIR156-OE,MIR408-OEand NIP plants under 10 μM IAA treatment. The red arrow indicates primary roots. Bar = 1 cm.KPrimary root length, adventitious root number and the length of three longest first-order crown roots in 2-week-old WT (ZH11),MIR156-OE, MIR408-OE/MIR156-OE,MIR408-OEand NIP plants under 10 μM IAA treatment. Error bars indicate SD (Tukey’s honestly significant difference,P< 0.05).LRepresentative phenotype of seedling roots of 2-week-old WT (ZH11),ipa1, MIR408-OE/ipa1and a negative plant used for crossing withoutMIR408-OE(CK/ipa1) under 10 μM IAA treatment. The red arrow indicates primary roots. Bar = 1 cm.MPrimary root length, adventitious root number and the length of three longest first-order crown roots in 2-week-old WT (ZH11),ipa1, MIR408-OE/ipa1and CK/ipa1plants under 10 μM IAA treatment. Error bars indicate SD (Tukey’s honestly significant difference,P< 0.05). Source data underlying (C,E–G,I,K,M) are provided as a Source Data file. 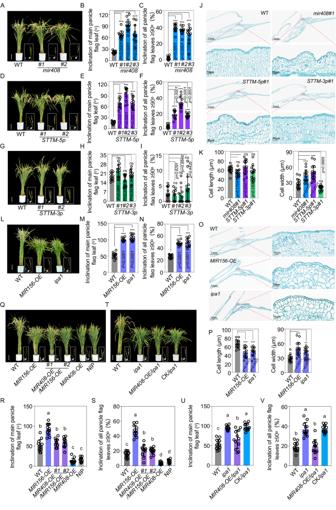Fig. 6: miR156-IPA1-miR408-5p-IAA30circuit regulates rice leaf inclination. Phenotypic observations ofmir408(A),STTM-5p(D) andSTTM-3p(G) and respective WT plants (Bars = 10 cm). Boxed regions are enlarged to the performance of flag leaves with panicles (Bars = 1 cm). White arrows indicate the lamina joints. Inclination of flag leaves on the main stem with panicles inmir408(B),STTM-5p(E) andSTTM-3p(H) and respective WT plants. Angles of flag leaf at 40 days after heading were measured and data are presented as means ± SD (standard deviation,n= 12). Statistical analysis was conducted by using Multiple comparisons test (***P< 0.001; ns not significant). The ratio of flag leaves with angle≥90°from all flag leaves on stems with panicles inmir408(C),STTM-5p(F) andSTTM-3p(I) and respective WT plants. Statistical analysis was executed by using Multiple comparisons test (***P< 0.001; ns not significant).JLongitudinal section of the adaxial region of the lamina joint in WT,mir408,STTM-5pandSTTM-3pflag leaves at 40 days after heading. The marked regions in red color were magnified to highlight the differences.KCell length and cell width of adaxial parenchyma cells of lamina joint in WT,mir408,STTM-5pandSTTM-3pplants. The fourth layer parenchyma cells at the adaxial side were calculated and statistically analyzed by Multiple comparisons test (***P< 0.001; ns not significant).LTypical plant phenotypes of WT (ZH11),miR156-OEtransgenic plants andipa1mutants (Bars = 10 cm). Boxed regions are enlarged to the performance of flag leaves with panicles (Bars = 1 cm). White arrows indicate the lamina joints.MInclination of flag leaf on the main stem with panicle in WT (ZH11),miR156-OEandipa1plants.NThe ratio of flag leaves with angle≥90°from all flag leaves on stems with panicles in WT (ZH11),miR156-OEandipa1plants.OLongitudinal section of the adaxial region of the lamina joint in WT (ZH11),miR156-OEandipa1flag leaves at 40 days after heading.PCell length and cell width of adaxial parenchyma cells of lamina joint in WT (ZH11),miR156-OEandipa1plants. Phenotypic comparisons in WT (ZH11),miR156-OE, miR408-OE/miR156-OE,miR408-OE, NIP plants (Q) and in WT (ZH11),ipa1, MIR408-OE/ipa1and CK/ipa1plants (T). Inclination of flag leaf on the main stem with panicle in WT (ZH11),miR156-OE, miR408-OE/miR156-OE,miR408-OE, NIP plants (R) and in WT (ZH11),ipa1, MIR408-OE/ipa1and CK/ipa1plants (U). The ratio of flag leaves with angle ≥90° from all flag leaves on stems with panicles in WT (ZH11),miR156-OE, miR408-OE/miR156-OE,miR408-OE, NIP plants (S) and in WT (ZH11),ipa1, MIR408-OE/ipa1and CK/ipa1plants (V). Source data underlying (B,C,E,F,H,I,K,M,N,P,R,S,UandV) are provided as a Source Data file. 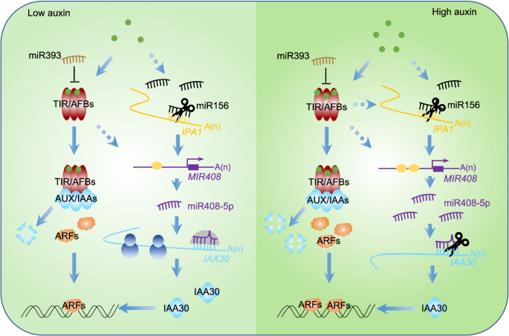Fig. 7: Working model of auxin signaling involving miR408-5p regulation in rice. Compared with that in low auxin environment, rice in high auxin condition represses miR156 and promotes more association of IPA1 withMIR408cis-element to trigger higher accumulations of mature miR408-5p, thereby leading to switch miR408-5p action from translation repression to mRNA cleavage. In addition to a higher contribution from canonical receptor-mediated auxin signaling, more robust regulation ofIAA30by miR408-5p in rice through mRNA cleavage results in an enhanced auxin response in a high than in a low auxin environment. The LUC images were taken by the imaging device (Tanon 5200) and the LUC signals were measured by GloMax Luminometer System (Promega, USA) and calculated by LUC/REN ratio. Yeast one-hybrid assays The coding sequence of IPA1 was amplified and subcloned into pGADT7 (Clontech). IAA30 promoter regions P1 (−1287 to −1264 bp before precursor), P2 (−558 to −414 bp before precursor), P3 (−425 to −108 bp before precursor), P4 (−151 to 4 bp before precursor) were amplified and subcloned into pAbAi vector. The resulting constructs were then transformed into yeast strain Y1HGold. The yeast transformants were cultured on dropout (-Leu) medium containing 150–300 ng/ml Aureobasidin A (AbA) for 3 days before observation. The assay was performed with three replicates. Leaf angle measurement and cytological analysis Leaf lamina joints with 1 cm sections of the flag leaf and sheath of the main tiller were cut 40 days after heading and photographed. Leaf angle was calculated by 180° minus the angle between sheath and leaf using a semicircular instrument for at least 12 leaf angles of individual plants. For cytological section analysis, the leaf lamina joints were fixed in FAA solution (40% ethanol, 5% acetic acid, and 12.5% formaldehyde in water) for 24 h and then dehydrated in a graded ethanol series and xylene-ethanol solution. Samples were embedded in paraffin for 1 day, then sections were deparaffinized in xylene, hydrated via a graded ethanol series, and stained by Fast GreenFCF after a cut into small pieces. The extra stain was rinsed, and sections were re-dehydrated by a graded ethanol series and microscopically observed. Cell numbers, length and width were calculated by ImageJ software. Immunoblot quantification analysis Quantification of immunoblots was conducted according to the band intensities of Flag-IAA30 and Actin as a loading control for total lysates, which were measured with Image J . Relative band intensities were then calculated using the ratio of IAA30/Actin for each immunoblot. All immunoblot experiments were performed at least three times, essentially with the same conclusions. Reporting summary Further information on research design is available in the Nature Portfolio Reporting Summary linked to this article.